Targeting bacteria via iminoboronate chemistry of amine-presenting lipids Synthetic molecules that target specific lipids serve as powerful tools for understanding membrane biology and may also enable new applications in biotechnology and medicine. For example, selective recognition of bacterial lipids may give rise to novel antibiotics, as well as diagnostic methods for bacterial infection. Currently known lipid-binding molecules primarily rely on noncovalent interactions to achieve lipid selectivity. Here we show that targeted recognition of lipids can be realized by selectively modifying the lipid of interest via covalent bond formation. Specifically, we report an unnatural amino acid that preferentially labels amine-presenting lipids via iminoboronate formation under physiological conditions. By targeting phosphatidylethanolamine and lysylphosphatidylglycerol, the two lipids enriched on bacterial cell surfaces, the iminoboronate chemistry allows potent labelling of Gram-positive bacteria even in the presence of 10% serum, while bypassing mammalian cells and Gram-negative bacteria. The covalent strategy for lipid recognition should be extendable to other important membrane lipids. It is increasingly clear that membrane lipids do not merely provide a physical barrier for a cell; instead they play active roles in regulating numerous processes in cell physiology and disease [1] . To support the diverse functions of a membrane, the composite lipids, while maintaining the common feature of amphiphilicity, do vary in their chemical structures to give a complex lipidome ( Fig. 1a ) [2] , [3] . The lipid composition of a membrane has significant ramifications in biology. For example, it is well known that the plasma membranes of bacterial and mammalian cells display distinct compositions of lipids: while a mammalian cell membrane primarily consists of phosphatidylcholine (PC) and sphingomyelin (SM), bacterial cells display highly enriched phosphatidylethanolamine (PE) and phosphatidylglycerol (PG) [4] , [5] . In addition, some bacterial species present a lysine-modified PG (Lys-PG, Fig. 1a ) in high percentages as a resistance mechanism to cationic antibiotics [6] . Synthetic molecules that specifically target bacterial lipids may give rise to new imaging methods of bacterial infection, as well as novel solutions to the antibiotic-resistance problem. The critical importance of lipids also manifests in the subcellular distribution of certain lipids in mammalian cells, a change of which may alter the homeostasis of important signalling proteins [7] , [8] . To further elucidate the diverse roles of membrane lipids, it is highly desirable to have molecular probes that specifically target a lipid of interest as well. Currently known lipid-targeting agents, which are primarily lipid-binding proteins and their synthetic mimetics, achieve lipid recognition by employing networks of noncovalent interactions, such as hydrogen bonds and salt bridges [9] , [10] . It remains to be seen whether membrane lipids can be selectively recognized by covalently targeting their unique chemical structure and reactivity with synthetic molecules. 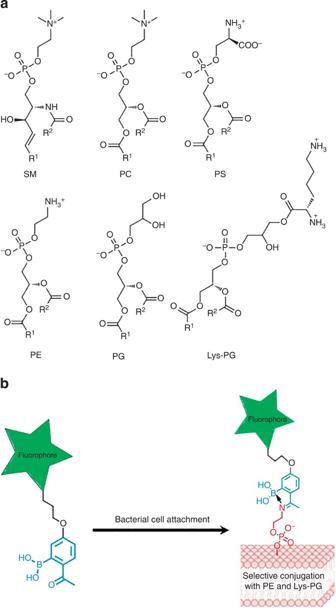Figure 1: Covalent recognition of membrane lipids. (a) Structures of the major membrane lipids from mamallian (sphingomyelin (SM) and phosphatidylcholine (PC)) and bacterial (phosphatidylethanolamine (PE), phosphatidylglycerol (PG), lysylphosphatidylglycerol (Lys-PG)) cells. PE and phosphatidylserine (PS) exist in mammalian cells as minority lipids. (b) Illustration of the iminoboronate chemistry for targeting PE on bacterial cell surfaces. Figure 1: Covalent recognition of membrane lipids. ( a ) Structures of the major membrane lipids from mamallian (sphingomyelin (SM) and phosphatidylcholine (PC)) and bacterial (phosphatidylethanolamine (PE), phosphatidylglycerol (PG), lysylphosphatidylglycerol (Lys-PG)) cells. PE and phosphatidylserine (PS) exist in mammalian cells as minority lipids. ( b ) Illustration of the iminoboronate chemistry for targeting PE on bacterial cell surfaces. Full size image In this contribution, we report the design and synthesis of an unnatural amino acid that selectively conjugates with amine-presenting lipids via formation of iminoboronates. By targeting the membrane lipids enriched in bacterial cells, namely PE and Lys-PG, the iminoboronate chemistry allows highly selective labelling of bacteria over mammalian cells. Design and synthesis of AB1 The two major bacterial lipids, PE and Lys-PG, differ from their mammalian counterparts (PC and SM) by the presence of primary amino groups. We postulated that these nucleophilic amines could be captured by a 2-acetylphenylboronic acid (2-APBA) motif to form an iminoboronate ( Fig. 1b ). Although theoretically possible, amines in biology milieu only forms a Schiff base with simple ketones at high concentrations [11] . For example, the association constant of acetone and glycine was reported to be 3.3 × 10 −3 M −1 . Usually, the imine formation is trapped with a reduction step for biological applications [12] . With the ortho boronic acid group serving as an electron trap, the 2-APBA motif conjugates with an amine much more readily to give an iminoboronate [13] , [14] , [15] , [16] , [17] . Importantly, the reaction proceeds under physiological conditions and in a reversible manner. Furthermore, an iminoboronate conjugate can exchange with other amines to allow for thermodynamic control of the final iminoboronate formation ( Supplementary Fig. 1 ) [15] . These features make the iminoboronate chemistry particularly suitable for facilitating molecular recognition in biological systems. To test our hypothesis, we have designed and synthesized a novel unnatural amino acid (AB1, Fig. 2 ) that presents a 2-APBA motif as its side chain. We envisioned that the amino-acid scaffold should allow the 2-APBA motif to be readily conjugated to fluorescent labels or other functional peptides. The synthetic route of AB1 is summarized in Fig. 2 . Briefly, with 2′,4′-dihydroxy acetophenone 1 as the starting material, regioselective alkylation of the 4′-OH followed by triflate protection of the 2′-OH yielded 3 with an overall 81% yield. By taking advantage of the powerful thiol-ene chemistry [18] , compound 3 was conjugated to two cysteine derivatives, respectively, to give the protected amino acids 4 and 7 in high yields. The key transformation of our synthesis is the Miyaura borylation [19] , which converts the triflate to the Bpin moiety. In our hands, rigorous control of temperature was critical to the success of the borylation step: the reaction did not initiate below 95 °C and prolonged heating at higher temperatures caused the complete loss of the Bpin moiety to give the protodeboronated product, a protected AB2 (ref. 20 ). With optimized conditions, the Bpin moiety was introduced with 70–80% yield. Fortuitously, with the boronic acid moiety eliminated, AB2 served as a perfect negative control for AB1 in the following membrane-binding studies. 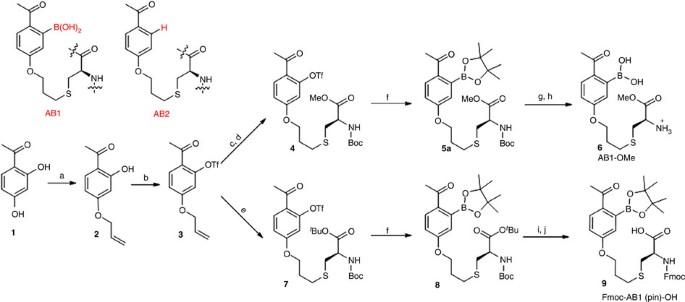Figure 2: Synthesis of AB1 and its derivatives. (a) Allyl bromide, K2CO3, NaI, acetone, 81%. (b) (CF3SO2)2O, Et3N, DCM, 95%. (c) Cys-OMe, DMPA, MeOH, ~365 nm ultraviolet irradiation. (d) Boc anhydride, Na2CO3, THF/H2O, 80% over two steps. (e) Boc-Cys-OtBu, DMPA, MeOH, ~365 nm ultraviolet irradiation, 75%. (f) Pd(dppf)Cl2/dppf, B2Pin2, KOAc, dioxane, ~70–80%. (g) 40% TFA in DCM. (h) diethanolamine, 1 N HCl, 74% over two steps. (i) 60% TFA in DCM. (j) Fmoc-OSu, Na2CO3, THF/H2O, 81% over two steps. DCM, dichloromethane; DMPA, 2,2-dimethoxy-2-phenylacetophenone; THF, tetrahydrofuran; TFA, trifluoroacetic acid. Figure 2: Synthesis of AB1 and its derivatives. (a) Allyl bromide, K 2 CO 3 , NaI, acetone, 81%. (b) (CF 3 SO 2 ) 2 O, Et 3 N, DCM, 95%. (c) Cys-OMe, DMPA, MeOH, ~365 nm ultraviolet irradiation. (d) Boc anhydride, Na 2 CO 3 , THF/H 2 O, 80% over two steps. (e) Boc-Cys-OtBu, DMPA, MeOH, ~365 nm ultraviolet irradiation, 75%. (f) Pd(dppf)Cl 2 /dppf, B 2 Pin 2 , KOAc, dioxane, ~70–80%. (g) 40% TFA in DCM. (h) diethanolamine, 1 N HCl, 74% over two steps. (i) 60% TFA in DCM. (j) Fmoc-OSu, Na 2 CO 3 , THF/H 2 O, 81% over two steps. DCM, dichloromethane; DMPA, 2,2-dimethoxy-2-phenylacetophenone; THF, tetrahydrofuran; TFA, trifluoroacetic acid. Full size image AB1 selectively conjugates with PE and Lys-PG The use of cysteine methyl ester (Cys-OMe) in the thiol-ene coupling step yielded the AB1 methyl ester (AB1-OMe, Fig. 2 ), which can be readily labelled with amine-reactive fluorophores. To assess the binding propensity towards different lipids, a fluorescein isothiocyanate-labelled AB1 methyl ester (Fl-AB1-OMe) was tested against lipid vesicles of varied composition. Specifically, 100nm-sized vesicles were prepared with PC alone or with 40% guest lipids including PE, PS, PG and Lys-PG. The fluorescence anisotropy values of Fl-AB1-OMe were recorded with increasing concentrations of lipids and the data are summarized in Fig. 3a . Interestingly, significant anisotropy increases were observed only with vesicles that present PE and Lys-PG, with other vesicle compositions eliciting marginal changes of anisotropy. Specifically, the presence of PG or PS did not induce more AB1 binding than PC-alone, showcasing the unique reactivity of PE and Lys-PG towards AB1. The lack of PS labelling by AB1 is perhaps surprising given that PS does display an amino group. This is presumably because the amino group of PS, in comparison to that of PE, is sterically more challenging for iminoboronate formation. This observation is consistent with a recent report, in which 2-APBA was found to preferentially react with lysine side chains over the main chain amino group [17] . Importantly, in contrast to Fl-AB1-OMe, Fl-AB2-OMe did not show significant association with the PC/PE or PC/Lys-PG vesicles ( Fig. 3b ), highlighting the importance of the boronic acid moiety in AB1 binding into vesicles. 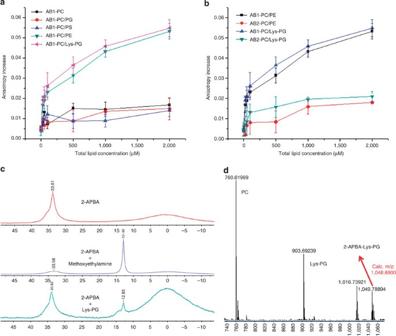Figure 3: Iminoboronate formation on synthetic vesicles. (a) Binding curves of Fl-AB1-OMe to lipid vesicles highlighting its selectivity for PE and Lys-PG. (b) Comparison of Fl-AB1-OMe and Fl-AB2-OMe for lipid binding showcasing the critical importance of the boronic acid moiety in vesicle association. All data points were measured with triplicate samples, from which error bars (s.e.m.) were generated. (c)11B-NMR spectra of 2-APBA (2-acetylphenylboronic acid) and its conjugates with methoxyethylamine and Lys-PG. The peaks around 13 p.p.m. correspond to the iminoboronates and the broad peaks around 0 p.p.m. originate from the NMR tube. (d) Mass-spec analysis of the iminoboronate conjugation of 2-APBA to PC/Lys-PG vesicles. The specific lipids used are POPC (1-palmitoyl-2-oleoylphosphatidylcholine) and Lys-DOPG (lysyl 1,2-dioleoylphosphatidylglycerol). 2-APBA-Lys-PG denotes the iminoboronate conjugate of 2-APBA and Lys-DOPG. Figure 3: Iminoboronate formation on synthetic vesicles. ( a ) Binding curves of Fl-AB1-OMe to lipid vesicles highlighting its selectivity for PE and Lys-PG. ( b ) Comparison of Fl-AB1-OMe and Fl-AB2-OMe for lipid binding showcasing the critical importance of the boronic acid moiety in vesicle association. All data points were measured with triplicate samples, from which error bars (s.e.m.) were generated. ( c ) 11 B-NMR spectra of 2-APBA (2-acetylphenylboronic acid) and its conjugates with methoxyethylamine and Lys-PG. The peaks around 13 p.p.m. correspond to the iminoboronates and the broad peaks around 0 p.p.m. originate from the NMR tube. ( d ) Mass-spec analysis of the iminoboronate conjugation of 2-APBA to PC/Lys-PG vesicles. The specific lipids used are POPC (1-palmitoyl-2-oleoylphosphatidylcholine) and Lys-DOPG (lysyl 1,2-dioleoylphosphatidylglycerol). 2-APBA-Lys-PG denotes the iminoboronate conjugate of 2-APBA and Lys-DOPG. Full size image To further validate the binding mechanism, we directly characterized the postulated iminoboronate conjugate of Lys-PG. Briefly, the PC/Lys-PG vesicles were treated with 2-APBA, the ‘warhead’ structure of AB1. Then the mixture was lyophilized, redissolved in CDCl 3 /CD 3 OD (2:1) and subjected to 11 B-NMR and mass spectrometry analysis. The 11 B-NMR spectrum of the treated lipids displays a peak around 13 p.p.m. as expected for iminoboronate structures ( Fig. 3c ). The mass-spec data clearly present the molecular ions that correspond to the 2-APBA adduct of Lys-PG ( Fig. 3d ). Further, mass-spec analysis also reveals the iminoboronate conjugate of Lys-PG and an AB1-presenting peptide ( Supplementary Fig. 2 ). These data consistently support the iminoboronate mechanism for the association of AB1 with lipid membranes. The iminoboronate mechanism predicts that the iminoboronate formation between AB1 and lipids can be inhibited by the presence lysine and lysine-presenting proteins. Indeed, lysine and bovine serum albumin (BSA) were found to disrupt the association of AB1 and PC/PE vesicle with an IC 50 of ~0.3 mM and 5 μM, respectively ( Supplementary Fig. 3 ). It is interesting to note that BSA at 5 μM gives ~0.3 mM in lysine concentration given that BSA has a total of 59 lysine residues. In a later section, we will present strategies that minimize the protein interference of AB1-labelling lipids. AB1 selectively labels Gram-positive bacteria Encouraged by the model membrane studies, we sought to investigate the potential of AB1 in staining bacterial cells. Three strains of bacteria, including B. subtilis (American Type Culture Collection (ATCC) 663) , S. aureus (ATCC 6538) and E. coli (BL 21), were selected as the initial set, which are known to have PE and/or Lys-PG as the major lipids of their plasma membranes [4] , [5] , [6] . The bacterial cells were stained with an Alexa Fluor 488 (AF488)-labelled AB1-OMe, which was chosen for cell studies because of the superior brightness and stability of the fluorophore. At concentrations below 1 μM, little fluorescence staining of the cells was observed with AF488-AB1-OMe. With higher concentrations, a quick washing procedure was included to minimize background fluorescence, after which the samples were immediately examined under an epi-fluorescence microscope ( Fig. 4a ). With wash, AF488-AB1-OMe effectively stained the two Gram-positive bacteria ( B. subtilis and S. aureus ) at ≥100 μM concentrations. In sharp contrast, the Gram-negative E. coli showed no fluorescence staining at all. As a negative control, AF488-AB2-OMe failed to stain any of the bacterial strains under the same conditions ( Supplementary Fig. 4 ), showcasing the critical importance of the boronic acid moiety for bacteria labelling by AB1. The labelling can be inhibited by the addition of lysine ( Supplementary Fig. 5 ) or BSA ( Supplementary Fig. 6 ), lending further support to the iminoboronate mechanism of conjugation. To gain more mechanistic insights, we analyzed the lipid extract of the S. aureus cells treated with 2-APBA: the 11 B-NMR spectrum clearly revealed the characteristic peak (~13 p.p.m.) for iminoboronates ( Supplementary Fig. 7 ), although our trials with mass-spec failed to identify the expected conjugates directly. 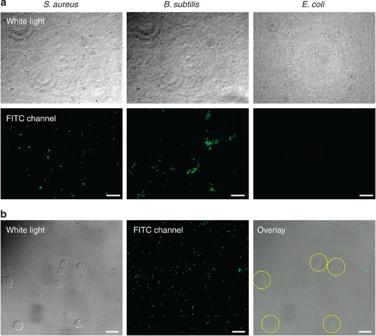Figure 4: Assessing the selectivity of AB1 for various cell types. (a) Microscopic images of three bacterial strains stained with 200 μM AF488-AB1-OMe (scale bar, 10 μm), showing that the AB1 derivative readily labels Gram-positive bacteria, but not Gram-negatives. (b) Confocal microscopic images of a mixed cell culture consisting ofS. aureusand Jurkat lymphocytes stained with 100 μM AF488-AB1-OMe (scale bar, 25 μm). The Jurkat cells are highlighted by the yellow circles on the overlay image. These results collectively demonstrate the superb selectivity of AB1 for Gram-positive bacteria. FITC, fluorescein isothiocyanate. Figure 4: Assessing the selectivity of AB1 for various cell types. ( a ) Microscopic images of three bacterial strains stained with 200 μM AF488-AB1-OMe (scale bar, 10 μm), showing that the AB1 derivative readily labels Gram-positive bacteria, but not Gram-negatives. ( b ) Confocal microscopic images of a mixed cell culture consisting of S. aureus and Jurkat lymphocytes stained with 100 μM AF488-AB1-OMe (scale bar, 25 μm). The Jurkat cells are highlighted by the yellow circles on the overlay image. These results collectively demonstrate the superb selectivity of AB1 for Gram-positive bacteria. FITC, fluorescein isothiocyanate. Full size image The failure of AB1 to stain E. coli is consistent with the fact that the outer membrane of E. coli does not have PE or Lys-PG. It further indicates that AF488-AB1-OMe is unable to permeate through the outer membrane to reach the plasma membrane, where PE does exist. Consistent with the membrane impermeability of AF488-AB1-OMe, we found that the fluorescence staining of S. aureus could be rapidly and completely washed away with a pH 5.0 buffer ( Supplementary Fig. 8 ). The failure of E. coli staining suggests that AB1 does not label cell surface proteins under the experimental conditions, the exact mechanism of which remains to be further investigated. One possible explanation is that certain features of the membrane, such as local membrane curvature [21] , create kinetic traps for AB1. Supporting this hypothesis, we found that, after the initial washing step, the cell-bound AB1 molecules dissociate from the cell very slowly at neutral pH ( Supplementary Fig. 8 ). Another possibility is that the number of surface proteins might be significantly smaller than that of lipids; consequently labelled surface proteins afford negligible fluorescence in comparison to labelled lipids. We further assessed the selectivity of AB1 for bacteria over mammalian cells. Excitingly, when a co-culture of Jurkat lymphocytes and S. aureus cells was treated with AF488-AB1-OMe and analysed under a confocal microscope, strong fluorescence staining was observed for S. aureus cells, whereas the Jurkat cells were minimally labelled ( Fig. 4b ). Similar to the result of E. coli staining, the lack of Jurkat cell staining also indicates that AF488-AB1-OMe does not conjugate with cell surface proteins under our experimental conditions. Further, as we learned from the bacterial staining experiments, AF488-AB1-OMe is membrane impermeable, which precludes labelling of intracellular targets. Finally and importantly, there are few AB1-reactive lipids on the outer surface of Jurkat cells: a mammalian cell does not unusually produce Lys-PG. Although PE can account for up to 20% of the total lipids of a mammalian cell [1] , it is primarily confined to the cytosolic leaflet and therefore not available at the cell surface either [7] . AB1 synergizes with cationic peptides for potent bacteria labelling Despite the remarkable selectivity for Gram-positive bacteria, simple AB1 derivatives like AF488-AB1-OMe suffer from the high concentrations needed to achieve effective bacteria labelling. Furthermore, dictated by the mechanism of iminoboronate formation, AB1 derivatives are expected to react with lysine and lysine residues of various proteins [17] , which in turn inhibit the association of AB1 with membranes. For example, BSA was found to inhibit the bacterial cell labelling by AF488-AB1-OMe with an apparent IC 50 of ~1.5 mg ml −1 (~22 μM). At 10 mg ml −1 concentration, BSA resulted in ~90% reduction of the fluorescence staining of the AF488-AB1-OMe-treated S. aureus cells ( Supplementary Fig. 6 ). We surmised that these problems could be resolved by conjugating AB1 to a directing functionality to bacterial cells. Towards this end, we have synthesized AB1 in its properly protected form (Fmoc-AB1(pin)-OH, Fig. 2 ) for solid-phase peptide synthesis, which should allow facile conjugation of AB1 to a variety of peptides or peptidomimetics that can serve as bacteria-directing motifs. Given that bacterial cells are known to be enriched with negatively charged lipids, such as PG and cardiolipin, we thought to employ cationic peptides to direct AB1 to bacterial cell surfaces [22] , [23] . A small group of peptides were synthesized to incorporate AB1 as the C-terminal residue ( Fig. 5a ). The bacteria-targeting elements we tested include single cationic residues Lys and Arg, as well as a polycationic peptide Hlys [24] , [25] with the sequence of RYWVAWRNR. Hlys was reported to give a minimal inhibitory concentration of 24 μM against S. aureus , yet minimal haemolytic activity [24] . In addition, we chose Hlys because of its small size and the absence of lysine residues, which could in principle form an intramolecular iminoboronate with AB1. Nevertheless, we did not see intramolecular iminoboronate formation with the peptide K-AB1 ( Supplementary Fig. 9 ). This lack of intramolecular conjugation is possibly due to the potential steric constraint that results from the fact that lysine and AB1 are contiguous in sequence. An analogous observation was recently reported for a cysteine-mediated macrocyclization with adjacent residues [26] . A control peptide (G-AB1) was also synthesized that incorporates a glycine instead of cationic motifs. All peptides were synthesized with an N-terminal cysteine so that they can be easily labelled with AF488-C5-maleimide ( Fig. 5a ). 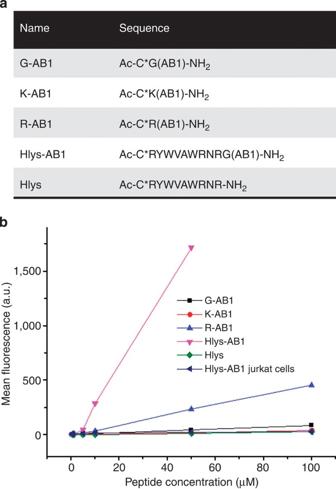Figure 5: Synergizing covalent and noncovalent interactions for bacteria targeting. (a) Sequences of AB1-presenting peptides, where C* represents a cysteine labelled with AF488-C5-maleimide. (b) Concentration profiles ofS. aureuscell staining by the AB1-presenting peptides. All samples were prepared with the washing step right before analysis. The data for Jurkat cell staining with Hlys-AB1 were included to show its superb bacterial selectivity. The flow cytometry experiments were performed twice, which gave consistent results. One set of the data is presented herein. Figure 5: Synergizing covalent and noncovalent interactions for bacteria targeting. ( a ) Sequences of AB1-presenting peptides, where C* represents a cysteine labelled with AF488-C5-maleimide. ( b ) Concentration profiles of S. aureus cell staining by the AB1-presenting peptides. All samples were prepared with the washing step right before analysis. The data for Jurkat cell staining with Hlys-AB1 were included to show its superb bacterial selectivity. The flow cytometry experiments were performed twice, which gave consistent results. One set of the data is presented herein. Full size image The fluorescently labelled peptides were first assessed via flow cytometry analysis of the S. aureus cells stained with peptides at varied concentrations ( Fig. 5b and Supplementary Fig. 10 ). The control peptide G-AB1 was only able to give a small fluorescence increase even at concentrations up to 100 μM. This is consistent with the fact that high concentrations of AF488-AB1-OMe are needed to achieve effective staining of bacterial cells. Conjugating AB1 to a lysine (K-AB1) did not improve, and perhaps even compromised AB1’s association with S. aureus . In contrast, conjugation to an arginine (R-AB1) significantly enhanced the cell labelling. This contrasting results for K-AB1 and R-AB1 can be rationalized by the fact that an arginine side chain can afford stronger interaction with phospholipids than a lysine [27] . The AB1 conjugate with the polycationic peptide Hlys (Hlys-AB1) afforded a dramatic improvement of its potency for bacterial cell staining. For example, at 50 μM, Hlys-AB1 afforded a mean fluorescence intensity 8 times higher than that of R-AB1 and over 40 times better than G-AB1. In contrast, Hlys alone did not afford any fluorescence staining of S. aureus cells ( Fig. 5b ), again highlighting the critical importance of the AB1 moiety that covalently conjugates with the membrane lipids of bacterial cells. Importantly, Jurkat cells were not stained by Hlys-AB1 even with the highest concentration tested ( Fig. 5b ). Finally, we note that under our experimental conditions Hlys-AB1 caused marginal reduction of the viability of the bacterial cells ( Supplementary Fig. 11 ), indicating the Hlys-enhanced staining is not due to the appearance of dying or dead bacterial cells, which may stain with AB1 differently. With much improved potency, we assessed Hlys-AB1 for bacteria labelling at nanomolar concentrations, with which the washing procedure is no longer necessary. The microscopic images show that, without wash, Hlys-AB1 effectively stained S. aureus cells at concentrations of 100 nM or higher ( Fig. 6 and Supplementary Fig. 12 ). The confocal images revealed the cell envelope localization of the Hlys-AB1 ( Supplementary Fig. 13 ), as expected for its membrane-targeting mechanism. Including the washing step in sample preparation resulted in approximately sevenfold reduction of the fluorescence staining of the cells ( Supplementary Fig. 14 ). This is perhaps not surprising considering the reversible nature of the iminoboronate chemistry. Importantly, Hlys alone did not label the S. aureus cells under the same conditions ( Fig. 6a ), highlighting the critical importance of the AB1 moiety for the Hlys-AB1 staining of bacterial cells. Excitingly, Hlys-AB1 remained highly selective for Gram-positive bacteria under the no-wash conditions: the peptide failed to afford any fluorescence staining for the Gram-negative E. coli ( Fig. 6b ), as well as the Jurkat lymphocytes ( Fig. 6e ). 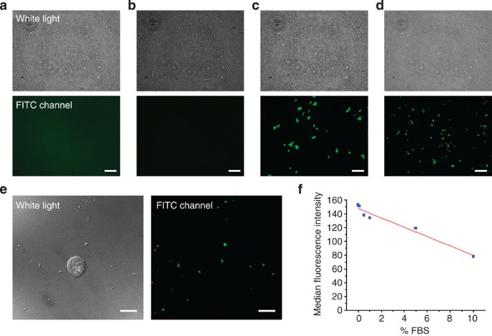Figure 6: Bacterial labelling with submicromolar concentrations of Hlys-AB1. (a)S. aureuscells treated with 0.5 μM Hlys as a negative control. (b)E. colitreated with 0.5 μM Hlys-AB1. (c)S. aureuscells stained with 0.5 μM Hlys-AB1. (d)S. aureuscells stained with 0.5 μM Hlys-AB1 in the presence of 10% FBS. (e) Confocal images of aS. aureusand Jurkat cell mixture stained with 0.5 μM Hlys-AB1. (f) FBS inhibition ofS. aureuscell staining by Hlys-AB1 analysed via flow cytometry. 0.2 μM Hlys-AB1 was used for this experiment. The median fluorescence (y-axis) appears to give a linear relationship against the percentage of FBS (x-axis). The flow cytometry experiments were performed twice, which gave consistent results. One set of the data is presented. FITC, fluorescein isothiocyanate. Figure 6: Bacterial labelling with submicromolar concentrations of Hlys-AB1. ( a ) S. aureus cells treated with 0.5 μM Hlys as a negative control. ( b ) E. coli treated with 0.5 μM Hlys-AB1. ( c ) S. aureus cells stained with 0.5 μM Hlys-AB1. ( d ) S. aureus cells stained with 0.5 μM Hlys-AB1 in the presence of 10% FBS. ( e ) Confocal images of a S. aureus and Jurkat cell mixture stained with 0.5 μM Hlys-AB1. ( f ) FBS inhibition of S. aureus cell staining by Hlys-AB1 analysed via flow cytometry. 0.2 μM Hlys-AB1 was used for this experiment. The median fluorescence ( y -axis) appears to give a linear relationship against the percentage of FBS ( x -axis). The flow cytometry experiments were performed twice, which gave consistent results. One set of the data is presented. FITC, fluorescein isothiocyanate. Full size image With the design of Hlys-AB1, the antimicrobial peptide Hlys is expected to selectively bind bacterial cell membranes and direct AB1 to covalently label PE or Lys-PG on bacterial cells. We hypothesized that this synergistic mechanism would not only improve the potency for bacteria labelling, but also minimize the protein interference of the iminoboronate chemistry. To prove this hypothesis, we assessed the inhibitory effect of fetal bovine serum (FBS) on the bacterial staining of Hlys-AB1. S. aureus cells were treated with Hlys-AB1 in presence of FBS at varied concentrations and the samples were analyzed with fluorescence microscopy and flow cytometry ( Fig. 6d,f ). The results show that, even with 10% FBS, submicromolar concentrations of Hlys-AB1 readily allowed the visualization of S. aureus cells under a fluorescence microscope ( Fig. 6d ), although reduced brightness was observed in comparison to the cells treated without FBS. Flow cytometry analysis yielded consistent results with microscopy: the presence of 10% FBS elicited ~30% reduction of the median fluorescence of the stained S. aureus cells ( Fig. 6f ). Again we attribute the much reduced protein interference of Hlys-AB1 to the synergy of covalent (AB1) and noncovalent (cationic peptide) mechanisms for bacterial cell targeting. The high potency and bacterial selectivity makes Hlys-AB1 potentially useful for targeting bacteria in blood serum or further in living organisms. To summarize, we have demonstrated that the two major membrane lipids of bacterial cells, namely PE and Lys-PG, can be selectively targeted by synthetic molecules that induce formation of iminoboronate structures. Specifically, we have synthesized an unnatural amino acid (dubbed AB1) that displays a 2-APBA motif and can therefore conjugate with primary amines to form iminoboronates. By targeting the differential abundance and accessibility of Lys-PG and PE on cell surfaces, a fluorophore-labelled AB1 effectively stains Gram-positive bacteria ( B. subtilis and S. aureus ), bypassing Gram-negative bacteria and mammalian cells. Conjugating AB1 to cationic peptides greatly enhances its potency for bacteria labelling and importantly minimizes the interference of serum proteins to its bacterial association. Specifically, a hybrid peptide Hlys-AB1 was found to label S. aureus cells at nanomolar concentrations even in the presence of 10% FBS. Nature primarily employs noncovalent mechanisms, such as hydrogen bonding, to achieve specific molecular recognition. Covalent chemistry has been largely avoided in targeting biomolecules of interest as irreversibility could result in modification of unintended targets and consequently toxicity [28] , [29] . However, reversible covalent chemistry circumvents this problem and should be able to complement the noncovalent mechanisms for molecular recognition. Among the limited number of examples, Wells and co-workers reported a strategy for protein ligand discovery that utilizes reversible disulfide chemistry to target reactive cysteines [30] . More recently, a group of nitrile modified acrylamides was reported by the Taunton group that reacts with cysteines of a protein kinase in a rapidly reversible manner [31] . In addition to targeting thiols, various boronic acid-presenting structures have been developed to target certain carbohydrates via reversible boronic ester formation [32] , [33] . Our work presented here, together with some recent publications by others [16] , [17] , expands the reversible covalent chemistry toolbox for targeting biological amines. Although the iminoboronate chemistry was previously shown to label purified proteins [17] and aminosugars [16] , the selectivity over other biomolecules has not been addressed. In comparison, our work here clearly demonstrates the applicability of the iminoboronate chemistry in complex biological systems (for example, bacteria labelling in the presence of blood serum). It is highly desirable, yet challenging to differentiate various membrane lipids. A recent report [34] describes the covalent modification of mammalian aminophospholipids (PE and PS) on cell surfaces with an amine reactive reagent named sulfo-NHS-biotin, which allows the capture and quantification of externalized aminophospholipids. The nonselective reactivity of this reagent towards amines precludes its use in complex biological milieu. With the goal of better understanding lipid biology, a number of chemically modified lipids have been developed to display bioorthogonal reacting groups [35] , [36] , [37] , [38] . Once incorporated into a membrane, lipids as such can be selectively labelled to reveal their subcellular distribution and homeostasis behaviour. However, these synthetic lipid probes are not known to afford specificity for bacterial cells. A recent report by Dumont et al . describes the metabolic incorporation of an azide-modified sugar into lipopolysaccharide [39] , which enables fluorescence labelling of Gram-negative bacteria without genetic modification. Our work differs from these previous reports because the AB1 derivatives selectively target natural endogenous lipids of Gram-positive bacteria. For the purpose of bacterial detection, this contribution complements the elegant work by Dumont and co-workers, which is limited to selected Gram-negative bacteria. The results of in vitro characterization presented here clearly demonstrate the superb bacteria selectivity, as well as the minimal serum interference, of AB1 and derivatives. Ongoing research in our lab seeks to further improve the potency of the AB1 derivatives for fast and more efficient labelling of bacterial cells, as well as to improve their stability towards proteolytic degradation. Our future research will evaluate the potential of optimized AB1 derivatives for biomedical applications, such as detecting bacteria in blood samples or imaging bacterial infection in animal models [40] . Finally, we submit that the covalent strategy for molecular recognition should be extendable to other important lipids of biological membranes. Research towards this end is also currently underway. Materials and instrumentation Chemical reagents for small molecule and peptide synthesis were purchased from various vendors and used as received. The phospholipids were purchased from Avanti Polar Lipids (Alabaster, Al). PBS buffer, DMEM/high-glucose media, RPMI 1640 media and penicillin/streptomycin were purchased from Thermal Scientific. The Gram-positive bacteria ( B. subtilis (ATCC 663) and S. aureus (ATCC 6538)) were purchased from Microbiologics as lyophilized cell pellet. E. coli (BL 21) was a gift from the lab of Professor Mary F. Roberts at Boston College. NMR data of the small molecules were collected on a VNMRS 500 MHz NMR spectrometer. Mass spectrometry data were generated by using an Agilent 6230 LC TOF mass spectrometer. Peptide synthesis was carried out on a Tribute peptide synthesizer from Protein Technologies. The fluorescence anisotropy experiments were performed by using a SpectraMax M5 plate reader. Fluorescence images were taken on a Zeiss Axio Observer A1 inverted microscope. Confocal images were taken on the Leica SP5 confocal fluorescence microscope housed in the Biology Department of Boston College. Flow cytometry analyses were carried out on a BD FACSAria cell sorter also housed in the Biology Department of Boston College. Synthesis Details of the amino acid and peptide synthesis are provided as Supplementary Methods . Also presented in Supplementary Figs 15–25 are the NMR spectra of novel compounds, exemplary high-performance liquid chromatography traces of the fluorophore-labelled AB1 derivatives, and in Supplementary Table 1 are mass-spec data of the fluorophore-labelled amino acids and peptides. Binding assays with lipid vesicles Liposomes were prepared by dissolving and mixing the desired phospholipids in chloroform. After evaporating chloroform, the residue was suspended in 50 mM phosphate buffer, pH 7.4. The lipid suspensions were treated through 10 cycles of freeze-and-thaw process, and extruded 11 times through a membrane with pore size of 100 nm. The concentrations of liposome stocks were characterized via the Stewart Assay [41] . The size distribution of each vesicle sample was characterized with a dynamic light scattering instrument (DynaproTM NanoStar, Wyatt Technology Corp.). The diameter of all vesicles were found to fall into the narrow range of 100–120 nm. Lipid vesicles at varied concentrations (25, 50, 100, 500, 1,000, 2,000 μM total lipids) were incubated with 0.5 μM of Fl-AB1/2-OMe for 40 min in a phosphate buffer (50 mM Na·Pi, pH=7.4). Then the fluorescence anisotropy values of each sample were recorded. To correct for the interference of light scattering, the lipid binding data of fluorescein isothiocyanate-alaninamide were used for blank subtraction. All samples were measured in triplicates and the data were averaged to generate the binding curves. NMR and mass spectrometry characterization of iminoboronates The PC/Lys-PG (3:2) vesicles (200 μl, 2 mM total lipids) were incubated with 2-APBA (200 μl, 10 mM) and Ac-R-AB1-amide (200 μl, 2 mM), respectively, for 40 min. Then the mixtures were lyophilized and dissolved in CDCl 3 :CD 3 OD (2:1; 600 μl). The iminoboronate formation was confirmed by 11 B NMR and mass spectrometry. All the 11 B-NMR experiments were carried out with BF 3 as an external standard, the chemical shift of which was set at 0 p.p.m. BF 3 was not used as an internal standard because of its acidic nature, which might disrupt the iminoboronate conjugates. Bacterial cell culture and staining Bacterial staining experiments were performed against three strains: B. subtilis (ATCC 663), S. aureus (ATCC 6538) and E. coli (BL21). For each strain, bacterial cells from a single colony were grown overnight in LB broth at 37 °C with agitation. An aliquot was taken and diluted (1:50 for E. coli , 1:20 for B. subtilis , 1:200 for S. aureus ) in fresh broth and cultured for another ~3 h until the cells reached the mid-logarithmic phase (OD 600 ~0.5). Then the bacterial cell culture was diluted ten times and used immediately for small molecule labelling. For a typical labelling experiment, 100 μl of the diluted bacterial cell culture was spun down at 7,000 r.p.m. in a centrifuge tube (1.5 ml). The cells were washed once with 100 μl phosphate buffer (50 mM Na·Pi, pH=7.4), and then mixed with 100 μl solution of an AB1 derivative at desired concentrations. After 40 min incubation, the samples with low AB1 concentrations (≤1 μM) were directly analyzed. The samples with higher AB1 concentrations were subjected to a washing procedure: the cells were spun down at 7,000 r.p.m. and the supernatant was discarded. Then the cells were washed twice with the phosphate buffer (100 μl, 2 min incubation), after which the spun-down cells were re-suspended in 50 μl of the phosphate buffer for analysis. Mammalian cell culture and staining Jurkat cells were grown and maintained in RPMI 1640 media with 10% FBS and 1% penicillin/streptomycin at 37 °C, 5% CO 2 and passed for less than 50 generations. The cell viability and density was checked and counted daily by using 0.2 μM trypan blue as a viability testing dye on a haemocytometer. Before staining with a small molecule, the cells were cultured to a density of 1.5–2.0 × 10 6 cells per ml in a Corning cell culture flask (with vent cap). Small-molecule staining was carried out by a similar protocol as used for the bacterial cells except the speed of centrifugation (Jurkat cells were spun down at 200 r.c.f. (relative centrifugal force)). Samples with high AB1 concentrations (>1 μM) were washed right before analysis. Co-culture preparation For labelling with AF488-AB1-OMe, 500 μl of Jurkat (1.5~2.0 × 10 6 cells per ml) cells and 100 μl of S. aureus (2-3 × 10 8 cells per ml) were separately stained with 100 μM AF488-AB1-OMe in centrifuge tubes for 40 min. Then the Jurkat and S. aureus cells were spun down at 200 r.c.f. and 7,000 r.p.m., respectively. The supernatants were discarded and the cells were further washed twice with 100 μl of the phosphate buffer. Finally, the Jurkat and S. aureus cells were re-suspended in 50 μl of phosphate buffer and mixed together for imaging study. For the labelling experiment with Hlys-AB1, 500 μl of Jurkat (1.5~2.0 × 10 6 cells per ml) cells and 100 μl of S. aureus (2-3 × 10 8 cells per ml) were mixed. The mixture was incubated with 0.5 μM Hlys-AB1 for 40 min and then immediately subjected to microscopy analysis. Microscopic analysis of AB1-stained cells For epi-fluorescence microscopy, 5 μl of the bacterial cell suspension was dropped on a glass slide (Fisherfinest premium, 75 × 25 × 1 mm 3 ). A coverslip (Fisherbrand, 22 × 22 × 0.15 mm 3 ) was pressed down on the cell droplet to give a single layer of cells on the glass slides. White light and fluorescence images were taken on a Zeiss Axio Observer A1 inverted microscope equipped with a filter cube (488 nm excitation, 515–520 nm emission) suitable for detection of AF488 fluorescence. A Plan-NeoFluar × 100 oil objective from Zeiss was used to visualize the bacterial cells. All images were captured with the exposure time of 300 ms for AF488-labelled AB1 derivatives. All fluorescence images were processed following a fixed protocol with the software Fiji ImageJ [42] . For confocal analysis, 5 μl of cells were placed on a glass slide and a 22 × 22 × 1.5 Fisherbrand microscope cover glass was placed on top. Images were taken on a Leica SP5 confocal fluorescence microscope with filters that allowed detection of AF488 (488 nm excitation, 496–564 nm emission). A × 63 oil objective was used with an Argon laser at 10% laser power. Gain was adjusted to between 900 HV and 1,100 HV with an offset of −0.5%. The images were captured with the software LAS 2.6 and then processed with Fiji ImageJ [42] . Flow cytometry analysis of AB1 stained cells The samples were prepared and stained following the same protocol described for microscopy. The cells stained with sub-micromolar concentrations of Hlys-AB1 were analyzed without wash, while all other samples were subjected to the wash procedure right before analysis. The samples were analyzed on a BD FACSAria cell sorter (BD Biosciences). Data analysis was performed with FlowJo (Tree Star, Inc.), from which the median fluorescence intensities of the stained cells were extracted and plotted against AB1 concentration. For the protein inhibition experiments, the cell samples were prepared in the presence of BSA or FBS at desired concentrations before the addition of the AB1 compounds. The median fluorescence intensity of these cell samples was extracted and plotted against BSA or FBS concentration. How to cite this article: Bandyopadhyay, A. et al . Targeting bacteria via iminoboronate chemistry of amine-presenting lipids. Nat. Commun. 6:6561 doi: 10.1038/ncomms7561 (2015).